Freezing-in orientational disorder induces crossover from thermally-activated to temperature-independent transport in organic semiconductors The crystalline structure of organic materials dictates their physical properties, but while significant research effort is geared towards understanding structure–property relationships in such materials, the details remain unclear. Many organic crystals exhibit transitions in their electrical properties as a function of temperature. One example is the 1:1 charge-transfer complex trans -stilbene—2,3,5,6-tetrafluoro-7,7,8,8-tetracyanoquinodimethane. Here we show that the mobility and resistivity of this material undergo a transition from being thermally activated at temperatures above 235 K to being temperature independent at low temperatures. On the basis of our experimental and theoretical results, we attribute this behaviour to the presence of a glass-like transition and the accompanied freezing-in of orientational disorder of the stilbene molecule. Organic semiconductors have earned an increasing amount of research interest in the past decade due to their promise of viability in low-cost, large-area and flexible electronic applications [1] , [2] . Of particular interest are organic charge-transfer (CT) complexes; these are combinations of charge-donating (D) and charge-accepting (A) compounds that individually tend to be unipolar semiconductors, but that together can exhibit entirely different properties as a result of interactions between the donor and acceptor units. CT complexes are often subject to phase transitions as a function of temperature and pressure, resulting in changes in electrical properties at a critical temperature or pressure. Examples include metal-insulator transitions, neutral-ionic transitions, Peierls transitions and transitions to a ferroelectric state [3] , [4] , [5] , [6] , [7] , [8] , [9] , [10] , [11] , [12] , [13] . Historically, these complexes were of interest due to the prediction of room temperature superconductivity or metallic conductivity [14] ; more recently, they have proven to be an excellent medium for the study of novel application-oriented properties such as photoconductivity, tunable semiconductivity, ferroelectricity, magnetoresistance and field emission [3] , [4] , [15] , [16] , [17] , [18] , [19] , [20] , [21] , [22] , [23] , [24] , [25] , [26] . Such properties are highly coupled to the crystalline structure of these molecular solids. For example, BEDT-TTF TCNQ (where BEDT-TTF is the donor bis(ethylenedithio)tetrathiafulvalene and TCNQ is the acceptor 7,7,8,8-tetracyanoquinodimethane) can crystallize in either a mixed-stack motif (in which D and A molecules alternate in a linear stack) or a segregated-stack motif (in which D and A molecules form separate stacks). While the constituents of these polymorphs are represented in exactly the same ratio in both crystals, the mixed stack material is a semiconductor with a conductivity of 10 −6 Ω −1 cm −1 and a degree of charge transfer from the donor to the acceptor of q =0.2e, and the segregated-stack material is a metal with a conductivity of 10 1 Ω −1 cm −1 and a degree of charge transfer of q =0.5e [27] , [28] , [29] . In this article, we investigate the effect of thermally-induced static and dynamic structural modifications on the electronic and electrical properties of the CT complex composed of the donor trans -stilbene (STB; Fig. 1a,b ) and the acceptor 2,3,5,6-tetrafluoro-7,7,8,8-tetracyanoquinodimethane (F 4 TCNQ; Fig. 1c,d ) by using a combined experimental and theoretical approach. This binary crystal grows in a 1:1 ratio, crystallizes in a mixed-stack array along the a axis, and will be referred to as STB-F 4 TCNQ ( Fig. 1e,f ). We have discovered that it exhibits a crossover from temperature-independent to thermally-activated charge transport around 235 K. Similar transitions have been observed recently in a series of semiconducting polymers [30] , [31] and in the small-molecule organic semiconductor 6,13-bis-triisopropyl-silylethynyl pentacene (TIPS-pentacene) [32] , [33] . In STB-F 4 TCNQ, by combining a previous thermodynamic study on this system [34] with our X-ray diffraction (XRD) and optical measurements, we are able to attribute the observed behaviour to a glass-like transition. (Here the term ‘glass-like transition’ is adopted for a crystalline solid with some degrees of freedom frozen-in, as described in detail in other reports [35] , [36] , [37] , [38] , [39] , [40] , [41] .) This transition does not distort the crystal lattice, but is accompanied by the freezing-in of orientational disorder related to the torsional oscillation (libration) of the double bond connecting the C7 and C7a carbons in the STB molecule ( Fig. 1a ). Below the transition temperature, the librational motion is not sufficiently strong to mediate transitions between the states of different orientations. Librational motion is ubiquitous in organic semiconductors and was predicted to localize charge carriers in organic crystals [42] . While it was recently measured in TIPS-pentacene by thermal diffuse electron scattering [43] , this motion has been difficult to connect with experimental observations of a material’s electronic properties. Our results provide direct insight into the effect of libration on electrical properties of organic molecular crystals, and show that its change in amplitude can result in a crossover from thermally-activated to a temperature-independent charge transport. 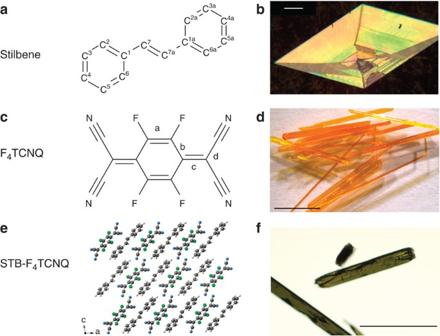Figure 1: The parent compounds and CT complex. (a) The donor stilbene skeletal structure with the atoms numbered to correspond with the crystallographic structure. (b) An optical image of a stilbene single crystal. Scale bar, 200 μm. (c) The skeletal structure of the acceptor F4TCNQ with bond lengths relevant to the calculation of degree of charge transfer labelled. (d) An optical image of F4TCNQ crystals. Scale bar, 5 mm. (e) The CT complex STB-F4TCNQ crystal structure that exhibits mixed stacking in theadirection. (f) An optical image of the STB-F4TCNQ crystal. Scale bar, 200 μm. Figure 1: The parent compounds and CT complex. ( a ) The donor stilbene skeletal structure with the atoms numbered to correspond with the crystallographic structure. ( b ) An optical image of a stilbene single crystal. Scale bar, 200 μm. ( c ) The skeletal structure of the acceptor F4TCNQ with bond lengths relevant to the calculation of degree of charge transfer labelled. ( d ) An optical image of F4TCNQ crystals. Scale bar, 5 mm. ( e ) The CT complex STB-F4TCNQ crystal structure that exhibits mixed stacking in the a direction. ( f ) An optical image of the STB-F4TCNQ crystal. Scale bar, 200 μm. Full size image Electrical properties We evaluate the electrical properties of the STB-F 4 TCNQ crystals by space-charge-limited current measurements. Although more than five crystals have been studied, we report here the results from one representative sample. The resistivity ( ρ ) is calculated from the ohmic region of the I – V (current–voltage) curve ( Fig. 2 ). 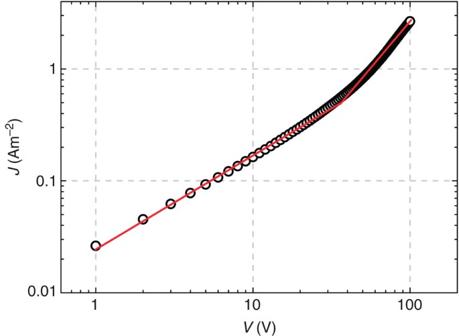Figure 2: Current–voltage characteristics of the STB-F4TCNQ crystal at 300 K. The slope in the low-voltage region is 0.85, and the slope in the high-voltage region is 2.01. The mobility ( μ ) is determined from the Mott–Gurney law, shown in equation (1), in the region where the current density, J SCLC , is proportional to V 2 : Figure 2: Current–voltage characteristics of the STB-F 4 TCNQ crystal at 300 K. The slope in the low-voltage region is 0.85, and the slope in the high-voltage region is 2.01. Full size image Here ε is the relative permittivity of the semiconductor (~3), ε 0 is the permittivity of free space and θ is the ratio of free charge carriers to total charge carriers (estimated to be 1, so the resulting mobility is a low estimation). As seen in Fig. 2 , the proportionality of J to V validates our use of both Ohm’s law and the Mott–Gurney law. The value of L / t (where L is the channel length and t is the thickness of the crystal) lies in the range 10–30, which is sufficiently low to validate our use of the Mott–Gurney law instead of the Guerst law [44] . 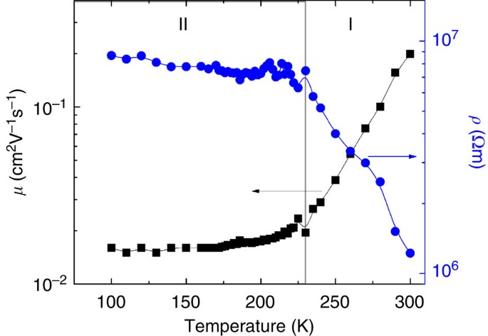Figure 3: The temperature dependence of the electrical characteristics of STB-F4TCNQ. The regions here are divided into I, where the transport is activated, and II, where the charge transport is temperature independent. Right axis, in blue: resistivity; left axis, in black: mobility. Figure 3 shows the resistivity (blue, right axis) and mobility (black, left axis) of STB-F 4 TCNQ as a function of temperature. The resistivity and the mobility each independently exhibit an inflection point around T =235 K. In the high-temperature region ( T >235 K), labelled I, the resistivity decreases with increasing temperature and the mobility is thermally activated with an activation energy E A =0.17 eV. At low temperatures ( T <235 K), marked by region II, the charge transport is temperature independent. Interestingly, Saito et al. [34] discovered a signature for a thermodynamic transition near the same temperature by measuring the heat capacity of STB-F 4 TCNQ as a function of temperature. It is therefore plausible to assume that both the change in electrical properties and the phase transition occur as a result of the same mechanism. Figure 3: The temperature dependence of the electrical characteristics of STB-F 4 TCNQ. The regions here are divided into I, where the transport is activated, and II, where the charge transport is temperature independent. Right axis, in blue: resistivity; left axis, in black: mobility. Full size image Crystal structure and electronic structure calculations To determine the nature of the transition, we first evaluate the crystal structure of the CT complex as a function of temperature using XRD. The temperature dependence of the lattice parameters of STB-F 4 TCNQ is plotted in Fig. 4a . At all investigated temperatures, the system crystallizes in the monoclinic space group P2 1 / n with two STB molecules and two F 4 TCNQ molecules per unit cell, each located at an inversion centre. The unit cell varies by the expected linear thermal expansion; 1.1% along all three unit cell axes and 3.1% for the total unit cell volume, with no evidence of the presence of a structural phase transition. Subsequently, based on the temperature-dependent structures, we have performed band structure calculations and evaluated the effective masses for both holes and electrons. The results are shown in Fig. 4b . Our calculations indicate that charge carriers have small effective masses only along the stacking directions, and that both hole and electron effective masses increase systematically with the increase in temperature. This dependence is consistent with the linear thermal expansion of the crystal. As the cell parameters increase, the distance between the STB and F 4 TCNQ molecules also increases. Consequently, the calculations suggest that the transfer integral ( t HL ) from the HOMO (highest occupied molecular orbital) of STB to the LUMO (lowest unoccupied molecular orbital) of the neighbouring F 4 TCNQ molecule decreases, resulting in an increase in the effective mass of both holes and electrons. Thus, the temperature dependence of the transfer integrals and effective masses derived from the static structure are not able to provide an explanation for the features observed at T =235 K in the electrical measurements. 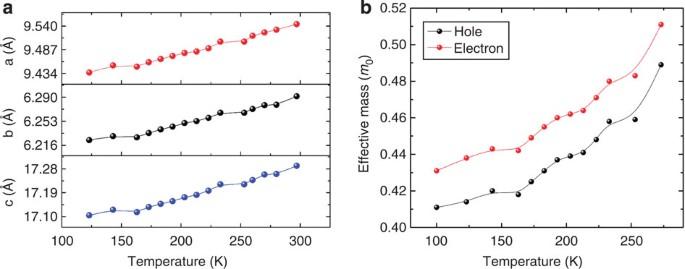Figure 4: The temperature dependence of properties of the CT complex. (a) The temperature dependence of the lattice parameters of STB-F4TCNQ. The lattice expansion is approximately linear with temperature. (b) The temperature dependence of the smallest component of the effective masses of holes and electrons as derived from band-structure calculations using the lattice parameters. Figure 4: The temperature dependence of properties of the CT complex. ( a ) The temperature dependence of the lattice parameters of STB-F 4 TCNQ. The lattice expansion is approximately linear with temperature. ( b ) The temperature dependence of the smallest component of the effective masses of holes and electrons as derived from band-structure calculations using the lattice parameters. Full size image Structure and thermodynamics Stilbene and related compounds have been the subject of intense research scrutiny for a number of years. In particular, static and dynamical disorders are known to play a significant role in the structure and properties of stilbene-containing compounds. Single-crystal XRD measurements of neat STB and the CT complex STB-TCNQ show that the STB molecule can adopt two orientations that are related to one another by a twofold rotation about the longest molecular axis [45] , [46] , [47] . The librational motion responsible for the interconversion between these two conformers can be viewed as a rotation of the central C=C stilbene moiety at fixed orientation of the benzene rings relative to the crystal lattice and is referred to as a pedal-like (crankshaft) motion. In the neat STB crystal, this motion results in an orientational disorder [48] , [49] . Variable-temperature structural studies indicate that this disorder is dynamic—that is, conformational interconversion is temperature dependent (and as a result the conformer populations are also), with the occupancy factor of the minor, energetically unfavourable conformer, decreasing as the temperature is lowered [45] , [48] , [49] , [50] . Below 170 K the pedal motion becomes inactive and thus the conformational disorder does not undergo any significant changes. The quantity of the minor conformer present at low temperatures can be increased by increasing the cooling rate, but always remains very low (<10% for flash-cooled crystals and <5% for slow-cooled crystals). Freezing of the conformational changes generates thermodynamic non-equilibrium states that persist below the transition temperature and represents a signature of a glass-like transition. The anomaly observed in calorimetry measurements at 170 K in STB was therefore attributed to this glass-like transition due to the freezing of the crankshaft motion [41] . It is important to note that the potential energy along the torsional coordinate connecting the two conformers of the stilbene molecules can be described by a double-well potential. The ensemble of systems described by such energy potentials are well-known models for glasses [51] , [52] . In addition to these observations in neat STB, thermodynamic transitions are also found in calorimetry measurements of CT complexes of STB—near 250 K in STB-TCNQ and near 240 K in STB-F 4 TCNQ (ref. 34 ). The transitions are similar in shape to that seen in neat stilbene and are therefore interpreted to be caused by the freezing of crankshaft motion; however, these materials have not been reported to exhibit temperature-dependent changes in conformer populations as stilbene does. In the CT complexes, while the C=C bond undergoes a similar librational motion, a quantitative analysis of the conformational interconversion was impossible under regular laboratory conditions. Indeed, our temperature-dependent STB-F 4 TCNQ structure determination indicates that the disorder is low and the population of the minor conformer is below 5% at all temperatures ( Supplementary Methods and Supplementary Fig. 1 ). Our results are in agreement with Saito et al. [34] who concluded based on the heat capacity measurements that while there is disorder present in STB-F 4 TCNQ, the population of the misoriented STB molecules is <10%, even at room temperature. The lack of significant changes in the crystal structure as the system passes through the transition temperature coupled with the stepped-like feature in the heat capacity measurements are clear signatures of a glass-type transition [35] , [36] . As a result, we believe that the mechanism for the observed transition in the transport properties of STB-F 4 TCNQ crystal is related to the transition into a glassy crystal, where the constituent STB molecules exhibit freezing of the orientational disorder and the thermal equilibrium is no longer attained. In addition, the existence of a glass-like transition is supported by a significant thermal history dependence, which is also observed in our measurements. Interestingly, the Fourier maps do show a qualitative difference in electron density surrounding the C=C bond below versus above the transition. At 143 K, below the transition temperature ( Fig. 5a ), the density appears constant throughout the molecule, with a slight excess of charge density around the centre ethylene bond, suggesting the presence of the minor conformer. Above the transition, at 253 K ( Fig. 5b ), the density shows a signature of the increasing torsional motion of this bond, in agreement with our observations described below. 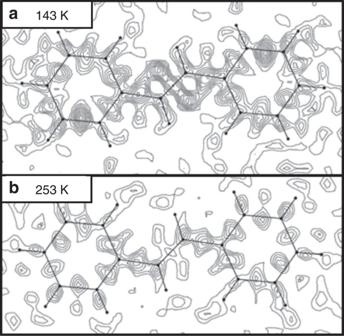Figure 5: Fourier difference maps above and below the transition temperatureT=235 K. (a) The Fourier difference map calculated for a temperature in region II (143 K). (b) The Fourier difference map calculated in region I (253 K). These show a redistribution of charge density around C7 and C7a. Positive contour lines were calculated at intervals of 0.05 Å. Figure 5: Fourier difference maps above and below the transition temperature T =235 K. ( a ) The Fourier difference map calculated for a temperature in region II (143 K). ( b ) The Fourier difference map calculated in region I (253 K). These show a redistribution of charge density around C7 and C7a. Positive contour lines were calculated at intervals of 0.05 Å. Full size image We gained further understanding of the dynamics of the central C=C bond in STB by analysing its change in length as a function of temperature. It is known that this bond can show apparent shrinking as a result of disorder or large-amplitude torsional motion [50] . In the present case, the C7=C7a ( Fig. 1a ) bond length gradually decreases with increasing temperature once the amplitude of the libration becomes large. Specifically, this bond length lies between the standard ethylene bond length of 1.34 Å and the fully conjugated benzene bond length of 1.39 Å at low temperatures, and it shortens to 1.322(6) Å at 273 K ( Fig. 6a ). Sato et al. [53] report a further shortened bond length of 1.315(4) Å at 293 K, also included in Fig. 6a . 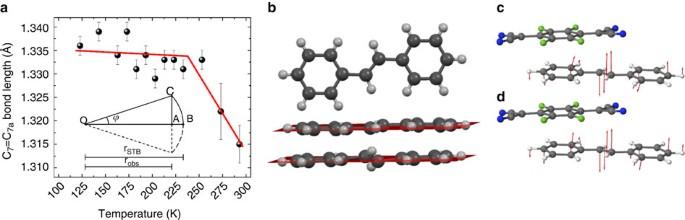Figure 6: Libration of the C7=C7a stilbene bond in STB-F4TCNQ. (a) The C7=C7a bond length is given as a function of temperature with the libration schematic as an inset. The error bars were calculated based on the s.d. of the bond lengths. (b) The oscillation of the C7 and C7a atoms above and below the plane formed by the benzene rings. (c) The eigendisplacements of the 279 cm−1phonon mode. (d) The eigendisplacements of the 285 cm−1phonon mode. Only one DA complex from the unit cell is shown. Figure 6b shows a schematic of the librational motion, with the C=C bond able to rotate above and below the plane created by the benzene rings. The calculations of the Γ-point phonons indicate that there are two vibrational modes with frequencies of 279 cm −1 ( Fig. 6c ) and 285 cm −1 ( Fig. 6d ) related to the libration of the STB bridge. As seen in Fig. 6c,d , the benzene rings are not involved in these modes—that is, these librations occur along the crankshaft trajectory. Assuming that the bond modification is due to librational motion, the root mean square libration amplitude, ϕ , can be obtained from the bond shortening by means of equation (2) [50] : Figure 6: Libration of the C7=C7a stilbene bond in STB-F 4 TCNQ. ( a ) The C7=C7a bond length is given as a function of temperature with the libration schematic as an inset. The error bars were calculated based on the s.d. of the bond lengths. ( b ) The oscillation of the C7 and C7a atoms above and below the plane formed by the benzene rings. ( c ) The eigendisplacements of the 279 cm −1 phonon mode. ( d ) The eigendisplacements of the 285 cm −1 phonon mode. Only one DA complex from the unit cell is shown. Full size image Here (see the inset in Fig. 6a ) r obs is the apparently shortened stilbene C7=C7a length as observed by diffraction and r stb is the expected C=C distance. Our calculations show that below the transition temperature the libration is small, reaching the detection limit, whereas above the transition it has an amplitude of ~10°, with the change taking place gradually, as the temperature is increased. This result shows for the first time a quantitative analysis of the temperature-dependent libration in organic crystals and supports the conclusion that the amplitude of this motion can directly affect charge transport in this class of materials. In addition to its effect on electrical properties of the STB-F 4 TCNQ crystals, libration significantly affects the partial degree of charge transfer ( q ) between the donor and acceptor molecules. In general, in organic CT complexes, the lattice expansion that occurs with increasing temperature yields larger intermolecular distances between the donor and acceptor species, resulting in weaker interactions between them and thus a lower q . The consequent decrease in t HL as described above is expected to lead to a decrease in the amount of charge transfer from STB to F 4 TCNQ in the ground state. Indeed, the lattice parameters and t HL follow the conventional trend; however, XRD, Raman and infrared (IR) spectroscopy indicate an increase in q with increasing temperature, as described below. Similar to its unfluorinated analogue, TCNQ, the bonds in F 4 TCNQ are sensitive to the value of q , allowing us to estimate this value based on bond lengths and vibrational frequencies. Thus, for our estimation of q from XRD measurements, we adapted the method reported for TCNQ-containing CT materials [54] . The bond lengths a and c ( Fig. 1a ) expand with increasing degree of charge transfer, while the bond lengths b and d shrink. The value for q can be calculated when these bond lengths are compared with the neutral F 4 TCNQ ( Supplementary Fig. 2 ), as in equation (3): Here bond lengths with the subscript ‘CT’ correspond to those of the acceptor within the CT complex STB-F 4 TCNQ ( Supplementary Fig. 3 ), while the bond lengths with subscripts of ‘N’ correspond to neutral F 4 TCNQ. Note that bond lengths for the neutral and CT F 4 TCNQ are compared at the same temperature so that thermal expansion does not affect the value for q . In Fig. 7 , we plot the results as a function of temperature, in black. Even though the structural changes follow the conventional behaviour in which the lattice expands with temperature, q nevertheless increases with temperature and mirrors the changes in the libration of the C7=C7a bond. This suggests that the libration increases the coupling between the donor and acceptor units and is responsible for the observed increase in q , in spite of the expansion of the unit cell. As Fig. 7 shows, q ~0 for T <235 K, where the libration is reduced in amplitude. As the temperature increases and the system passes through the transition, q increases to about 0.1e. 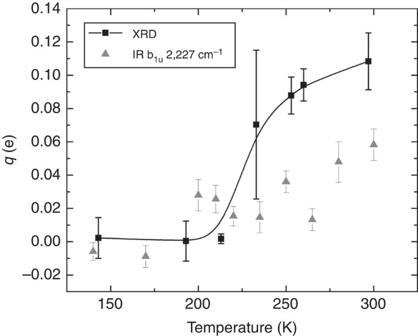Figure 7: Degree of charge transferqas a function of temperature. Values are derived from bond lengths (black, squares) and IR mode B1u(grey, triangles). All measurements show an increase in degree of charge transfer as a function of temperature. The error bars were calculated based on the s.d. of the bond lengths. Figure 7: Degree of charge transfer q as a function of temperature. Values are derived from bond lengths (black, squares) and IR mode B 1u (grey, triangles). All measurements show an increase in degree of charge transfer as a function of temperature. The error bars were calculated based on the s.d. of the bond lengths. Full size image This conclusion is also supported by our calculations of the degree of charge transfer using optical measurements ( Fig. 7 , in grey). It is known both experimentally and theoretically that, as for TCNQ, the frequencies of vibrations of the cyano groups of F 4 TCNQ vary linearly with the degree of charge transfer q [55] , [56] , [57] . There are four cyano-group vibrations; two are Raman active (A g and B 3g ) and two are infrared active (B 1u and B 2u ), with only the A g mode (2,225 cm −1 ) and the B 1u mode (2,227 cm −1 ) being experiementally observed ( Supplementary Methods , Supplementary Figs 4–7 ). The atoms in motion in these two vibrational modes are in close proximity to the surrounding molecules and may therefore be sensitive to the crystalline environment as well as to the degree of charge transfer [56] . The shift in frequency of the B 1u mode between the F 4 TCNQ neutral molecule and anion is 34 cm −1 , whereas the shift in frequency of the A g mode is only 6 cm −1 (ref. 56 ). Therefore, we use only the B 1u mode for the determination of the degree of charge transfer, shown in Fig. 7 . The temperature dependence of q as determined from the optical measurements shows the same behaviour as was determined from the XRD, although the values are somewhat smaller. The charge transfer is negligible at low temperatures and increases with temperature to a value not larger than 0.1 e at room temperature, in agreement with the XRD results. The Raman measurements of the A g mode ( Supplementary Methods ) agree with this finding. The observed increase in q with the increase of libration amplitude can be explained in terms of non-local (Peierls) electron–phonon coupling, which is the dependence of the transfer integrals on the displacements of the phonon modes [58] . The transfer integral, t HL computed as a function of the phonon displacements of the librational modes discussed above is shown in Fig. 8 . For small phonon displacements, t HL shows the expected linear behaviour [59] . However, for larger displacements, such as those expected above the transition temperature, t HL exhibits a significant non-linear increase. Therefore, the increase in the transfer integrals due to these librations surpasses the decrease related to the thermal expansion, leading to an overall increase of the t HL and, consequently, of the q with the increase in temperature. Our model thus aligns very well with the experimental observations. 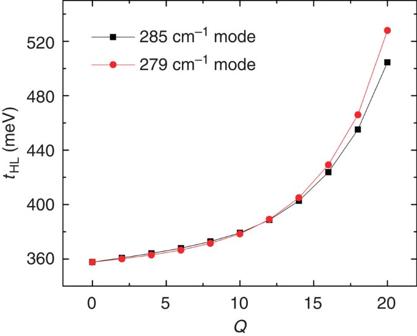Figure 8: Transfer integral dependence on the phonon displacements. The results for the 285 and 279 cm−1modes are indicated by black squares and red circles, respectively; the phonon displacements,Q, are given in dimensionless units. Figure 8: Transfer integral dependence on the phonon displacements. The results for the 285 and 279 cm −1 modes are indicated by black squares and red circles, respectively; the phonon displacements, Q , are given in dimensionless units. Full size image With a better understanding of the dynamics of the librational motion as a function of temperature, we are now able to describe the mechanism that can explain the evolution of the electrical properties of the STB-F 4 TCNQ crystals. One possible explanation for the crossover from tunnelling (and therefore temperature independence) at low temperatures to activated charge transport at higher temperatures invokes the interaction with local electron–phonon coupling (modulation of the site energies by vibrations), known as the Holstein small polaron model [58] , [60] . The Holstein polaron binding energy ( E pol ) of 0.14 eV estimated for STB-F 4 TCNQ in our previous study, however, results in an activation energy of ( E a ) of 0.07 eV ( E a = E pol /2), which is significantly smaller than the observed activation energy of 0.17 eV [22] . We note that the above estimation of the E pol and E a is based on the coupling with intramolecular vibrations only, that is, the contribution due to the electron–phonon interactions with intermolecular vibrations (lattice phonons) is neglected. Although the latter contribution to Holstein polaron binding energy in single-component systems is believed to be small, it may be different in the case of CT complexes. Therefore, while we cannot rule it out, we do not have at this point clear evidence that would support the implication of the Holstein-type electron–phonon coupling in the explanation of the observed crossover from temperature-independent to activated transport. A second possible explanation for the crossover could be related to the non-local electron–phonon coupling. This interaction can lead to an increase of the transfer integrals and subsequently to an enhancement of the transport properties (phonon assisted) [61] . At the same time, the Peierls-type coupling is a source of dynamical disorder and thus of charge localization [42] . If the former effect, which increases the mobility, were to dominate at high temperature, and the latter effect, which decreases the mobility, were to dominate at low temperatures, a crossover in the temperature dependence of the transport could result. Our previous results [22] indicate that the Peierls-type polaron binding energy in STB-F 4 TCNQ is smaller by an order of magnitude than the electronic coupling, and it is also much smaller than the experimental activation energy observed for the mobility. Therefore, we believe that the Peierls electron–phonon interaction is not the cause of the observed temperature dependence of the transport. We suggest that the observed transport behaviour is due to the double-well potential related to the librational motion of the center STB ethylene bond, which is also responsible for the glass-like transition in STB-F 4 TCNQ. At temperatures below the transition, the temperature-independent structural disorder is frozen-in and the transport can take place only via tunnelling of this manifold, therefore being temperature independent. At higher temperatures, when the interconversion motion is fast, a transition to temperature-activated hopping transport occurs. This proposed model is also supported by the measurements performed on analogue compounds, which exhibit orientational disorder at low temperatures: for both STB and STB-TCNQ, we observe a clear transition from a temperature-independent to activated transport at the same temperature where the glass transition occurs (see Supplementary Fig. 8 and Supplementary Discussion ). In conclusion, we show that the electrical characteristics of STB-F 4 TCNQ undergo a crossover from thermally activated at high temperatures to temperature independent below T =235 K. We attribute these changes to the presence of a glass-like transition, where a significant amount of orientational disorder of the STB molecule is frozen-in at low temperature upon reducing in amplitude of the libration of a molecular moiety within this molecule. When the libration is large, the structural disorder resulting from it yields a thermally-activated charge transport. At low temperatures, the transport is temperature independent and proceeds via tunnelling between the states created by the available conformers that generate the static orientational disorder. This transition has further implications within the class of organic CT complexes, as it affects the degree of charge transfer. These findings provide important insight into the effects that molecular dynamics—a ubiquitous feature in organic molecular materials—have on charge transport. Crystal growth The physical vapour transport crystal growth method was employed to grow single crystals when possible [62] , [63] . This method was successful for the growth of F 4 TCNQ single crystals. Here the commercial F 4 TCNQ (J&K Scientific or Sigma Aldrich) was heated to 220 °C under Argon flow. Platelet-like, yellow single crystals of a few millimetres in size formed in a quartz tube at the place where the temperature abruptly fell from 220 °C to room temperature. The vapour pressures of the donor and acceptor were too different to grow the STB-F 4 TCNQ crystals from the gas phase, so they were grown from solution instead. A few mg of trans-Stilbene (Sigma Aldrich) and F 4 TCNQ were weighed separately so that their molar masses were approximately 1:1. Each was dissolved in hot acetonitrile. The solutions were mixed and loosely covered to allow for slow solvent evaporation. Small, green, needle-like crystals of the 1:1 CT complex formed after 1–2 days. The crystals were washed with acetonitrile and filtered before use. We confirmed the structures of F 4 TCNQ and STB-F 4 TCNQ using single-crystal XRD measurements [53] . Structure determination Multiple data sets for single crystals of F 4 TCNQ and STB-F 4 TCNQ were collected over a temperature range from 123 to 297 K. Crystals of F 4 TCNQ are orthorhombic, space group Pbca with Z =4; crystals of STB-F 4 TCNQ are monoclinic, space group P2 1 / n (an alternate setting of P2 1 / c ) with Z =2 (formula units). A full-hemisphere of diffracted intensities (2,424 total 20-, 30- or 40-s frames with an ω scan width of 0.30°) was measured for each dataset using graphite-monochromated radiation ( λ =0.71073 Å) on a Bruker APEX CCD Single-Crystal Diffraction System. X-rays were provided by a fine-focus sealed X-ray tube operated at 50 kV and 30 mA. Lattice constants were determined with the Bruker APEX2 software package and integrated reflection intensities having 2 θ (( )≤60.00° were produced for each data set [64] . The structures were solved using ‘direct methods’ techniques and all stages of weighted full-matrix least-squares refinement were conducted using F o 2 data with the SHELXTL software package [65] . The resulting structural parameters for all data sets were refined to convergence using counter-weighted full-matrix least-squares techniques and structural models, which incorporated anisotropic thermal parameters for all non-hydrogen atoms. In STB-F 4 TCNQ, ring hydrogen atoms were included in the structural model as fixed atoms (using idealized sp 2 -hybridized geometry and C–H bond lengths of 0.93–0.95 Å) ‘riding’ on their respective carbon atoms. The hydrogen atom on the ethylene group was located from a difference Fourier map and was refined as an independent isotropic atom. The isotropic thermal parameters for the ring hydrogen atoms were fixed at a value 1.2 times the equivalent isotropic thermal parameter of the carbon atom to which they are covalently bonded. For the F 4 TCNQ and STB-F 4 TCNQ structures, totals of 91 and 158 parameters, respectively, were refined using no restraints. Difference electron density contour maps (F o −F c ) were generated using the Bruker programme XP. Full structural details for all structures are provided in the Supplementary Data 1 , as CIF files. Sample fabrication and electrical characterization Carbon paste (IPA base, Ted Pella) was painted on both ends of the long axis of the crystals to form a sandwich structure. I – V characteristics showed ohmic injection for this type of electrode. The crystals were placed on clean Si/SiO 2 to provide good electrical insulation. I – V characteristics were measured in vacuum (10 −6 Torr) and in the dark using an Agilent 4155C Semiconductor Parameter Analyzer. Current was measured while decreasing the temperature at 0.5 K min −1 ; measurements were taken every 10 K outside the region of the phase transition and with higher resolution around the phase transition. The crystals were stable through multiple rounds of measurement. IR spectroscopy Infrared absorption measurements were made using a Nicolet Nexus 670 FTIR spectrometer with a spectral range of 400–4,000 cm −1 . The small size of the crystals made single-crystal measurements impractical, so STB-F 4 TCNQ crystals were lightly crushed together and placed on a copper TEM grid with 54 micron grid-hole size. Temperature-dependent measurements were made using an MMR Technologies Joule-Thomson refrigerator over the temperature range 80–300 K. The spectrum as a function of temperature is shown in Supplementary Fig. 7 . Computational methodology Geometry optimizations of the crystal structures of STB-F 4 TCNQ at different temperatures were performed at the B3LYP/6-31G level of theory. During the optimizations, the unit cell parameters were kept fixed at the experimental values. A uniform 6 × 8 × 4 Monkhorst-Pack k-point grid was employed. Effective masses were obtained by diagonalizing the inverse effective mass tensor. Energy derivatives with respect to the k-point that form the tensor were evaluated using the finite-difference method with 0.01 Bohr −1 step. The Γ-point phonon modes were obtained using the finite-difference method with a 0.003 Å atomic displacement step. These calculations were carried out using the CRYSTAL09 package [66] . Transfer integrals (electronic couplings) between the HOMO of stilbene and the LUMO of F4TCNQ were calculated at the B3LYP/6-31G(d,p) level using a fragment orbital approach in combination with a basis set orthogonalization procedure [67] as implemented in the development version of the NWChem package [68] . How to cite this article: Goetz, K. P. et al. Freezing-in orientational disorder induces crossover from thermally activated to temperature-independent transport in organic semiconductors. Nat. Commun. 5:5642 doi: 10.1038/ncomms6642 (2014).